Modulating supramolecular binding of carbon dioxide in a redox-active porous metal-organic framework Hydrogen bonds dominate many chemical and biological processes, and chemical modification enables control and modulation of host–guest systems. Here we report a targeted modification of hydrogen bonding and its effect on guest binding in redox-active materials. MFM-300(V III ) {[V III 2 (OH) 2 (L)], LH 4 =biphenyl-3,3′,5,5′-tetracarboxylic acid} can be oxidized to isostructural MFM-300(V IV ), [V IV 2 O 2 (L)], in which deprotonation of the bridging hydroxyl groups occurs. MFM-300(V III ) shows the second highest CO 2 uptake capacity in metal-organic framework materials at 298 K and 1 bar (6.0 mmol g −1 ) and involves hydrogen bonding between the OH group of the host and the O-donor of CO 2 , which binds in an end-on manner, =1.863(1) Å. In contrast, CO 2 -loaded MFM-300(V IV ) shows CO 2 bound side-on to the oxy group and sandwiched between two phenyl groups involving a unique ···c.g. phenyl interaction [3.069(2), 3.146(3) Å]. The macroscopic packing of CO 2 in the pores is directly influenced by these primary binding sites. There is increasing interest in using porous materials for substrate binding, separation, storage, delivery and catalysis owing to their specific host–guest binding interactions [1] , [2] . Gaining molecular insights into these binding interactions is very important, but experimentally challenging. Firstly, the nature of host–guest binding is often within the regime of low-energy supramolecular contacts, and thus the guest molecules have great mobility in the pore and can be highly disordered [3] , [4] . For the study of hydrogen bonds in particular, the identification of structural and dynamic details has only been achieved via neutron scattering in exceptional cases [5] . Secondly, the porous nature of host materials leads to additional impediments for the in-depth investigation of host–guest systems, mostly due to the intrinsic structural disorder and overall lack of long-range order for certain types of porous materials (e.g., carbons, porous silica, large-pore zeolites) [6] , [7] . Design of a suitable host platform is the key to overcome these barriers to gain molecular information on the host–guest binding based upon multiple supramolecular contacts, particularly for hydrogen bonds. Metal-organic frameworks (MOFs) are an emerging class of porous materials showing highly crystalline structures and great promise for gas adsorption [8] , [9] . Built from metal ions/clusters and organic ligands, MOFs often exhibit high surface areas (up to ∼ 7,000 m 2 g −1 ) and, more importantly, tunable functional pore environments [10] , [11] , [12] . MOFs can readily incorporate desired functionality by judicious choice of metal nodes and/or organic linkers [13] , [14] , [15] . Post-synthetic modification, broadly defined as chemical derivatization of MOFs after their formation, can afford MOFs with additional functionalities that cannot be obtained by routine synthesis [16] , [17] . Fine-tuning of the supramolecular host–guest binding requires precise chemical modification to the functional groups on the MOF backbones. To govern the formation of hydrogen bonds in particular, such modification, involving removal/addition of protons, will trigger concurrent redox reactions to occur within the MOF hosts. Post-synthetic redox modification on MOFs without destroying/changing the pore structure, especially through a single-crystal to single-crystal transformation, rarely succeeds because of the changes in bond interactions which leads to collapse of the framework [18] , [19] , [20] . Redox modifications of MOFs have been reported for systems containing Fe II/III , V II/III/IV , Ti II/III/IV , Cu I/II and Cr II/III centres [21] , [22] . However, none of these MOF systems affords a pair of structural analogues (M n + and M n +1 -based MOF) as a platform for the direct investigation of guest binding. For example, MOF-74(Fe) features a hexagonal array of one-dimensional channels lined with co-ordinatively unsaturated Fe II centres [23] . The oxygen adsorption isotherm indicates that Fe II centres bind to O 2 preferentially over N 2 , which is attributed to a partial electron charge transfer from Fe II to O 2 . However, the Fe III -based MOF analogue cannot be isolated readily because, upon desorption of O 2 , the charge transfer is reversible. We report herein the synthesis of single crystals of a V III -based MOF, MFM-300(V III ) and its V IV isostructural counterpart, MFM-300(V IV ), which was obtained by oxidation of the V III precursor via a single-crystal to single-crystal transformation. These two materials show the same overall structural features with some differences in metal–ligand bond distances, but the main difference is conversion of V–(OH)–V in MFM-300(V III ) to V–O–V linkers in MFM-300(V IV ). This provides a unique platform to investigate the precise role of the OH group in the supramolecular binding of guest molecules. The binding of CO 2 has been thoroughly investigated in these two MOF systems via neutron diffraction and inelastic scattering, coupled with modelling. These experiments find that, surprisingly, the hydroxyl protons play a dominating role in the global binding of adsorbed CO 2 molecules in the pore, rather than just providing specific binding interactions to the localized CO 2 molecules nearby, as typically found in amine-functionalized MOFs [24] . Thus, as a result of the presence/absence of the hydroxyl proton, the binding and packing pattern for adsorbed CO 2 molecules in these two iso-structural MOFs are distinct. This study represents a unique analysis of the structural and dynamic characterization of hydrogen bonds (and other associated supramolecular interactions) that are stabilizing host–guest systems in the solid state. Synthesis and crystal structure of MFM-300(V III ) An oxygen-free hydrothermal reaction of VCl 3 , H 4 L (H 4 L=biphenyl-3,3′,5,5′-tetracarboxylic acid), HCl and water in the molar ratio of 6:1:1.5:1,600 at 210 °C for 3 days afforded MFM-300(V III )-solv, [V 2 (OH) 2 (L)]·6H 2 O, as a green microcrystalline material with a yield of ca. 90%. Single crystals of MFM-300(V III )-solv were obtained under acidic conditions (VCl 3 :H 4 L:HCl:water=16:1:53:11,000), which afforded dark green prism shaped crystals (0.5 × 0.2 × 0.2 mm; yield<5%) along with a large amount of re-crystallized organic ligand. It is likely that this highly acidic hydrothermal environment slows down the crystallization process of the MOF leading to slow growth of crystal nuclei into large crystals. Interestingly, synthesis of vanadium-based MOFs, especially in the single crystal form, has been very rarely reported [25] . It is also worth noting that oxygen-free conditions are necessary to prevent oxidation of V III centres during the hydrothermal process, and MFM-300(V III )-solv cannot be obtained in the presence of air/oxygen. 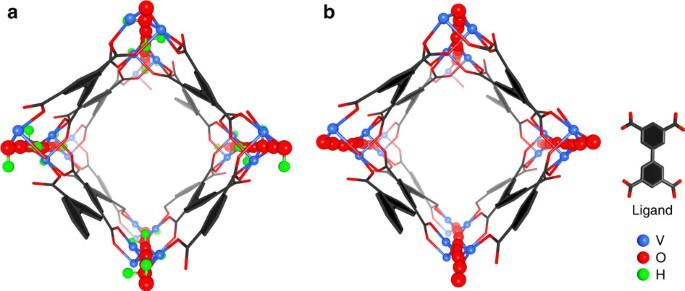Figure 1: Structures of MFM-300(V). Views of (a) MFM-300(VIII) and of (b) MFM-300(VIV). The pore size is∼6.7 × 6.7 Å for both MFM-300(VIII) and MFM-300(VIV) taking into consideration Van der Waals radii. The hydroxyl groups (green and red balls) in MFM-300(VIII) protrude into the channel, which change to O2-bridge (shown as red ball) in MFM-300(VIV). MFM-300(V III ) crystallizes in the space group I 4 1 22 and is isostructural to MFM-300(M) (M=Al, Ga, In, see Supplementary Table 1 for single crystal data) [26] , [27] , [28] . The V III centre shows octahedral coordination defined by four carboxylate oxygen atoms from the ligand [V–O=2.014(2) and 2.030(2) Å] and two oxygen atoms from two hydroxyl groups [V–O=1.948(2) Å] ( Fig. 1 ). Adjacent pairs of V III centres are bridged by two carboxylates and a μ 2 -hydroxyl group forming an extended chain of [V 2 (OH) 2 O 4 ] ∞ along the c axis. The ligands further bridge the vanadium hydroxyl chains to give a three-dimensional network with square-shaped channels decorated with hydroxyl groups. The cross-section of the channel is 6.7 × 6.7 Å taking Van der Waals radii into consideration. Guest water molecules in the channel can be readily removed by heating at 150 °C under vacuum for 5 h to give the desolvated material, MFM-300(V III ), as studied by in situ single crystal diffraction, which confirmed the retention of the framework structure and negligible residual electron density within the pore. The phase purity of MFM-300(VIII)-solv was confirmed by PXRD ( Supplementary Fig. 1 ). Figure 1: Structures of MFM-300(V). Views of ( a ) MFM-300(V III ) and of ( b ) MFM-300(V IV ). The pore size is ∼ 6.7 × 6.7 Å for both MFM-300(V III ) and MFM-300(V IV ) taking into consideration Van der Waals radii. The hydroxyl groups (green and red balls) in MFM-300(V III ) protrude into the channel, which change to O 2- bridge (shown as red ball) in MFM-300(V IV ). Full size image Post-synthetic oxidation to synthesize MFM-300(V IV ) The as-synthesized single crystals of MFM-300(V III ) changed colour from green to dark purple by heating at 150 °C under a flow of O 2 for 16 h to form MFM-300(V IV ), which were analysed by in situ single-crystal diffraction. MFM-300(V IV ) retains the space group I 4 1 22 and shows a slight contraction of the unit cell parameters (0.6% for a axis; 1.2% for c axis) with a similar channel size ( Table 1 ). The most significant structural change upon oxidation is that the V–O bond length involving the bridging oxygen reduces dramatically from 1.948(2) to 1.838(1) Å ( Table 1 ), which is between the typical bond distances for V III –O ( ∼ 1.95 Å) and V IV =O ( ∼ 1.65 Å) [21] . Detailed investigation of the crystal structure revealed no residual electron density close to the bridging V IV –O–V IV oxygen atom, indicating complete removal of the proton upon oxidation, which was further confirmed by neutron diffraction ( Supplementary Fig. 2 ). Bond valence sum calculations give a valence of 3.03 for MFM-300(V III ) and 3.96 for MFM-300(V IV ). Quantitative oxidation of vanadium centres on going from MFM-300(V III ) to MFM-300(V IV ) has been further confirmed by XPS spectroscopy, which shows increased binding energy for the V IV species ( Fig. 2 and Supplementary Fig. 3 ). IR spectroscopy confirms the disappearance in MFM-300(V IV ) of the ν O–H stretching mode of the hydroxyl group at 3,639 cm −1 observed in MFM-300(V III ) ( Fig. 6a and Supplementary Fig. 4 ). Thus, the post-synthetic oxidation leads to retention of the porous structures in these two materials, and therefore affords an excellent platform to compare the supramolecular binding of guest molecules as a function of the presence and absence of the hydroxyl protons within the channel. The oxidized material MFM-300(V IV ) can be reduced back to MFM-300(V III ) using Na 2 SO 3 in aqueous solution, with the colour of MFM-300(V IV ) changing from dark purple back to pale green, corresponding to the re-formation of MFM-300(V III ). PXRD data, however, confirm that some partial decomposition of the framework takes place under these conditions. Therefore, a quantitative reduction of MFM-300(V IV ) back to MFM-300(V III ) has not yet been achieved. Table 1 Unit cell parameters, bond lengths and bond valence calculations of MFM-300(V III ) and MFM-300(V IV ). 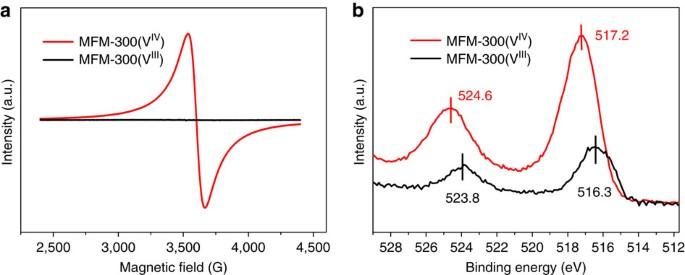Figure 2: Electron paramagnetic (EPR) resonance and X-ray photoelectron spectra (XPS). (a) Electron paramagnetic resonance (EPR) spectra and (b) X-ray photoelectron spectroscopy (XPS) of desolvated MFM-300(VIII) and MFM-300(VIV). The X-band (9.86 GHz) EPR spectra were collected at 293 K. MFM-300(VIII) is EPR silent under these conditions, consistent with VIII. MFM-300(VIV) has a strong EPR spectrum under the same conditions, giving a single resonance centred atg=1.955 (9.8661 GHz), consistent with VIV,d1(g<ge, the free electron value), with a peak-to-peak linewidth of ca. 130 G. Full size table Figure 2: Electron paramagnetic (EPR) resonance and X-ray photoelectron spectra (XPS). ( a ) Electron paramagnetic resonance (EPR) spectra and ( b ) X-ray photoelectron spectroscopy (XPS) of desolvated MFM-300(V III ) and MFM-300(V IV ). The X-band (9.86 GHz) EPR spectra were collected at 293 K. MFM-300(V III ) is EPR silent under these conditions, consistent with V III . MFM-300(V IV ) has a strong EPR spectrum under the same conditions, giving a single resonance centred at g =1.955 (9.8661 GHz), consistent with V IV , d 1 ( g < g e , the free electron value), with a peak-to-peak linewidth of ca. 130 G. Full size image Figure 6: Synchrotron micro-IR and inelastic neutron scattering (INS) spectra for MFM-300(V). Comparison of ( a ) the synchrotron micro-IR spectra and ( b ) INS spectra for bare MFM-300(V III ) and MFM-300(V IV ). IR and INS spectra offer vibrational information on the –OH stretching and deformation region, respectively, and are thus complementary. 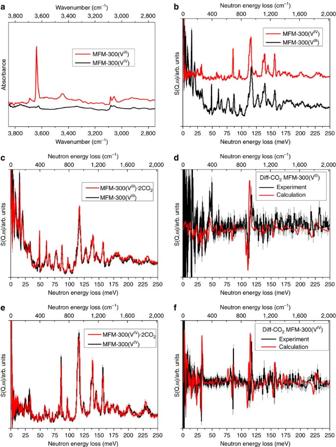Figure 6: Synchrotron micro-IR and inelastic neutron scattering (INS) spectra for MFM-300(V). Comparison of (a) the synchrotron micro-IR spectra and (b) INS spectra for bare MFM-300(VIII) and MFM-300(VIV). IR and INS spectra offer vibrational information on the –OH stretching and deformation region, respectively, and are thus complementary. (c) Comparison of the INS spectra for bare and CO2-loaded MFM-300(VIII); (d) difference spectra for both experiment and calculation showing changes of the H motion from the local MOF upon CO2binding in MFM-300(VIII). (e) Comparison of the INS spectra for bare and CO2-loaded MFM-300(VIV); (f) difference spectra for both experiment and calculation showing changes of the H motion from the local MOF upon CO2binding in MFM-300(VIV). Synchrotron IR and INS data were collected at 298 and 10 K, respectively. ( c ) Comparison of the INS spectra for bare and CO 2 -loaded MFM-300(V III ); ( d ) difference spectra for both experiment and calculation showing changes of the H motion from the local MOF upon CO 2 binding in MFM-300(V III ). ( e ) Comparison of the INS spectra for bare and CO 2 -loaded MFM-300(V IV ); ( f ) difference spectra for both experiment and calculation showing changes of the H motion from the local MOF upon CO 2 binding in MFM-300(V IV ). Synchrotron IR and INS data were collected at 298 and 10 K, respectively. Full size image It should be noted that the post-synthetic oxidation of MFM-300(V III ) is currently the exclusive way of obtaining MFM-300(V IV ); hydrothermal syntheses using VOSO 4 or VO 2 salts based upon conditions reported [25] for other vanadium-based MOFs failed thus far to produce MFM-300(V IV ) in our hands. Interestingly, MIL-47(V III ) and MIL-47(V IV ) also show one-dimensional channels constructed from [V 2 (OH) 2 O 4 ] ∞ chains bridged by terephthalate ligands [20] . MIL-47(V III ) and MIL-47(V IV ) can be synthesized directly from V III and V IV salts, respectively, but with considerable uncoordinated terephthalic acid encapsulated in the materials. Calcination of the as-synthesized complexes in air at 250 °C can effectively remove the free ligands to generate the corresponding activated materials. However, the V III centre was inevitably oxidized to V IV during calcination and the open form of MIL-47(V III ) could not be isolated until very recently when a new activation method based upon DMF extraction was developed that stabilized MIL-47(V III ) material. CO 2 and H 2 O adsorption isotherms confirm that MIL-47(V III ) and MIL-47(V IV ) exhibit significantly different degrees of framework flexibility upon guest inclusion, and therefore cannot be directly compared in terms of host–guest chemistry [29] . In contrast, MFM-300(V) incorporates a wine-rack framework connection tied together by strong cis -μ 2 -OH groups, resulting in isostructural, highly rigid and robust frameworks in both V III and V IV materials. Thermal gravimetric analysis (TGA) of MFM-300(V III )-solv shows that water can be fully removed at 200 o C under N 2 flow, and no further weight loss was observed to 450 °C when decomposition sets in ( Supplementary Fig. 5 ). In contrast, the TGA of MFM-300(V IV ) (prepared by heating under O 2 ) shows ∼ 2% weight loss before 120 °C, attributed to adsorbed moisture during sample transportation for TGA measurement. No further weight loss was observed to 490 °C, where the MOF decomposed. Electron paramagnetic resonance analysis To probe the change in oxidation state of V centres, electron paramagnetic resonance (EPR) studies at X-band (9.86 GHz) and room temperature were undertaken on MFM-300(V III ) and MFM-300(V IV ) ( Fig. 2 ). MFM-300(V III ) is EPR silent under these conditions, consistent with d 2 V III centre. In six-coordinate O h symmetry, the V III , d 2 ion has a 3 T 1g ground state. In lower symmetry, a 3 A state often results and spin–orbit coupling and gives rise to very large zero-field splitting (up to tens of cm −1 ) of the S =1 state (e.g., 5 cm −1 in [V(H 2 O) 6 ] 3+ ) [30] . Hence, most V III species are EPR silent at X-band where the microwave energy ( hν ) is only ca. 0.3 cm −1 . In contrast, MFM-300(V IV ) shows a strong EPR signal under the same conditions, giving a single resonance centred at g =1.955, consistent with V IV , d 1 ( g <g e , the free electron value), with a peak-to-peak linewidth of ca. 130 G. This broad linewidth is due to the exchange interactions in the V IV chains and results in the absence of any 51 V hyperfine resolution. Thus, EPR analysis confirms the change of oxidation state of V III to V IV in this system. Gas adsorption analysis N 2 isotherms at 77 K for both MFM-300(V) samples show no significant adsorption uptake, probably due to an activation diffusion effect at 77 K caused by the narrow pore channels. In contrast, low-pressure CO 2 isotherms of MFM-300(V III ) at ambient temperatures (273–303 K) show very high uptake capacities with a value of 8.6 mmol g −1 (37.8 wt%) recorded at 273 K and 1.0 bar ( Fig. 4 and Supplementary Figs 6 and 7 ), surpassing those of other MFM-300 analogues (7.0 mmol g −1 for MFM-300(Al) [26] , 2.86 mmol g −1 for MFM-300(Ga) [27] and 6.3 mmol g −1 for MFM-300(In) [28] ) under the same conditions. The CO 2 uptake of MFM-300(V III ) at 298 K and 1.0 bar is 6.0 mmol g −1 (26.4 wt%), comparable to the best-behaving materials such as MOF-74(Mg) or CPO-27(Mg) (26 ∼ 27.5 wt%) under the same conditions [31] . The CO 2 uptake in MFM-300(V IV ) is lower than that of its V III counterpart as a result of removal of the hydroxyl group from the pore. At 1.0 bar, the CO 2 uptake of MFM-300(V IV ) is 3.54 mmol g −1 (15.6 wt%) at 298 K and 6.56 mmol g −1 (28.9 wt%) at 273 K, a reduction of 41 and 25%, respectively, in comparison with MFM-300(V III ). Larger reductions in CO 2 uptake are observed at higher temperatures, consistent with reduced MOF-CO 2 binding strengths. The difference in CO 2 uptakes between these two materials is less pronounced with increasing pressure at a given temperature because the CO 2 intermolecular dipole interaction becomes more apparent at higher loadings. For example, at 273 K and 20 bar, the CO 2 uptake of MFM-300(V III ) and MFM-300(V IV ) were recorded to be 11.7 and 10.0 mmol g −1 , respectively, a difference of 14.5% ( Fig. 4d ). Analysis of the high-pressure CO 2 adsorption isotherm at 273 K by DFT/Monte-Carlo methods gives a surface area of 1,892 and 1,565 m 2 g −1 , a pore size distribution centred at 5.2 and 5.4 Å, and a cumulative pore volume of 0.490 and 0.481 cm 3 g −1 for MFM-300(V III ) and MFM-300(V IV ), respectively ( Fig. 4c and Supplementary Figs 8–13 ), confirming the microporous nature of these two materials. Interestingly, the slightly increased pore size (and wider distribution) of MFM-300(V IV ) is consistent with the deprotonation of the hydroxyl group in the channel, leading to decreased CO 2 uptake at low pressure. The pore size distribution analysis confirms a slightly smaller pore size than that measured from the X-ray single crystal structure consistent with the presence of activated diffusion in the gas adsorption isotherms. The narrow pore size can also afford enhanced overlapping potential to gas molecules, increasing the overall host–guest binding interactions, and the slightly reduced pore volume of MFM-300(V IV ) is responsible for its lower uptake capacity at high pressure in comparison with MFM-300(V III ). 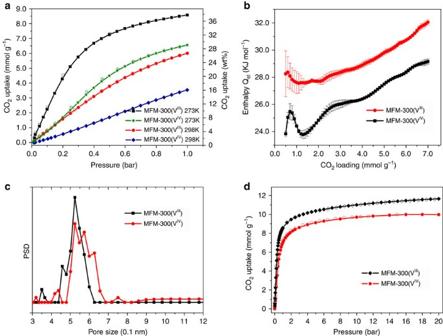Figure 4: View of the gas adsorption data. Figure 4: View of the gas adsorption data. (a) Comparison of the CO2adsorption isotherms for MFM-300(VIII) and MFM-300(VIV) at 273 and 298 K and 1.0 bar. (b) Variation of isosteric heat of adsorptionQstas a function of CO2uptake for MFM-300(VIII) and MFM-300(VIV) calculated using the van’t Hoff isochore on CO2adsorption isotherms measured at 273–303 K. Standard deviations are represented by error bars. (c) Comparison of the pore size distribution plots for MFM-300(VIII) and MFM-300(VIV), suggesting a slightly wider pore size in the latter material. (d) Comparison of the CO2adsorption isotherms for MFM-300(VIII) and MFM-300(VIV) at 273 K up to 20 bar. ( a ) Comparison of the CO 2 adsorption isotherms for MFM-300(V III ) and MFM-300(V IV ) at 273 and 298 K and 1.0 bar. ( b ) Variation of isosteric heat of adsorption Q st as a function of CO 2 uptake for MFM-300(V III ) and MFM-300(V IV ) calculated using the van’t Hoff isochore on CO 2 adsorption isotherms measured at 273–303 K. Standard deviations are represented by error bars. ( c ) Comparison of the pore size distribution plots for MFM-300(V III ) and MFM-300(V IV ), suggesting a slightly wider pore size in the latter material. ( d ) Comparison of the CO 2 adsorption isotherms for MFM-300(V III ) and MFM-300(V IV ) at 273 K up to 20 bar. Full size image The isosteric heat of adsorption ( Q st ) for CO 2 adsorption in MFM-300(V III ) (obtained using van’t Hoff Equation) lies in the range 27.5–28 kJ mol −1 for uptakes of 0.5–1.0 mmol g −1 and increases continuously thereafter to 32 kJ mol −1 at 7 mmol g −1 , which is slightly higher than that of MFM-300(Al) by ∼ 1.0 kJ mol −1 ( Fig. 4b ). In comparison, the Q st for MFM-300(V IV ) is 24 kJ mol −1 at low CO 2 coverage and increases steadily to 29 kJ mol −1 at 7 mmol g −1 , which is some ∼ 3 kJ mol −1 lower than that of MFM-300(V III ), confirming the presence of a weaker adsorbate–adsorbent binding interaction in MFM-300(V IV ). Nevertheless, the increasing trends of the variation of Q st plots are the same for these two materials, suggesting the presence of strong CO 2 –CO 2 interactions with increasing surface coverage in both materials. The binding energy of CO 2 in both MFM-300(V) materials has also been estimated by DFT calculations at a loading of 8.6 mmol g −1 (equivalent to 2 CO 2 /V). The stepwise calculation was carried out by (i) optimizing the structure of the bare MOF by finding the local potential energy minimum with the final potential energy E 1 ; (ii) optimizing the structure of the CO 2 -loaded MOF (2 CO 2 /V) with the final potential energy E 2 ; (iii) removing the MOF host and leaving the CO 2 molecules in the system to minimize the energy E 3 . The CO 2 binding energy (Δ E ), obtained by the calculation of Δ E = E 1 − E 2 + E 3 , was 34.9 and 29.7 kJ mol −1 for MFM-300(V III ) and MFM-300(V IV ), respectively, consistent with the Q st analysis and confirming a lower CO 2 -MOF binding strength in MFM-300(V IV ). Structural analysis by neutron powder diffraction In order to determine the binding sites of CO 2 within these two materials, neutron powder diffraction (NPD) experiments were carried out for CO 2 -loaded MFM-300(V III ) and MFM-300(V IV ) samples at 7 K. NPD data enabled full structural analysis via Rietveld refinement ( Supplementary Figs 14–17 and Supplementary Table 2 ), yielding the positions, orientations and occupancies of adsorbed CO 2 molecules within the materials. CO 2 -loaded MFM-300(V III ) retains the space group I 4 1 22 and two crystallographically independent CO 2 sites (I and II) were observed ( Fig. 5 ). Molecules CO 2 I are disordered with the respect to a two-fold rotation axis and are in an end-on mode interacting with the hydroxyl group with a distance of 1.863(1) Å ( Fig. 5 and Supplementary Fig. 18 ), shorter than that obtained for MFM-300(Al) (2.298(4) Å) by PXRD at 273 K (ref. 20 ). This suggests a stronger hydrogen bond between adsorbed CO 2 and the HO–V III group and probably reflects the difference in the acidity between the bridging Al–OH and V–OH groups. CO 2 II binds to the carboxylate oxygen atoms via a dipole interaction with distances ranging from 2.984(2) to 3.369(2) Å. Further dipole interactions were observed between adsorbed CO 2 molecules on sites I and II with intermolecular C I ···O II distance of 3.103(1) Å in a typical T-shape arrangement ( Fig. 5c ), comparable to that observed in dry ice (3.178(1) Å) [32] . Supplementary intermolecular π···π interactions are also observed between the CO 2 molecules at site II with a C II ···O II distance of 2.565(2) Å. 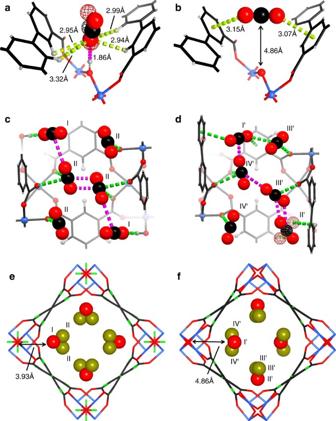Figure 5: Comparison of the crystal structures for CO 2 -loaded MFM-300(V III ) and MFM-300(V IV ) studied by NPD at 7 K. ( a ) Interactions of CO 2 molecule at site I with the hydroxyl and the –CH on phenyl groups in MFM-300(V III ). Figure 5: Comparison of the crystal structures for CO2-loaded MFM-300(VIII) and MFM-300(VIV) studied by NPD at 7 K. (a) Interactions of CO2molecule at site I with the hydroxyl and the –CH on phenyl groups in MFM-300(VIII). (b) 'Sandwiched' binding mode between CO2molecule on site I' with the phenyl groups in MFM-300(VIV). (c) CO2molecules at sites I and II within MFM-300(VIII) (disordered CO2on site I is shown in the averaged positions). Thedistances are in the range of 2.984(2) to 3.369(2) Å. The C···O distance between T-shape arranged CO2is 3.178(1) Å and that betweenπ–πinteracted CO2is 2.565(2) Å. (d) CO2molecules at sites I′ to IV′ within MFM-300(VIV). Thedistance is 2.666(2) Å. Thedistances are in the range of 2.843(2) to 3.057(2) Å. C···O distances between T-shape arranged CO2are in the range of 2.478(1) to 3.132(1) Å and that betweenπ–πinteracted CO2is 2.741(2) Å (carbon, black; hydrogen, light grey; oxygen, red; vanadium, light blue; interactions between CO2and frameworks are shown in green dashed line; interactions between adsorbed CO2molecules are shown in pink dashed line). (e) Binding sites for adsorbed CO2within MFM-300(VIII). (f) Binding sites for CO2within MFM-300(VIV) (red and dark yellow balls indicate the centre of the corresponding binding site). ( b ) 'Sandwiched' binding mode between CO 2 molecule on site I' with the phenyl groups in MFM-300(V IV ). ( c ) CO 2 molecules at sites I and II within MFM-300(V III ) (disordered CO 2 on site I is shown in the averaged positions). The distances are in the range of 2.984(2) to 3.369(2) Å. The C···O distance between T-shape arranged CO 2 is 3.178(1) Å and that between π – π interacted CO 2 is 2.565(2) Å. ( d ) CO 2 molecules at sites I′ to IV′ within MFM-300(V IV ). The distance is 2.666(2) Å. The distances are in the range of 2.843(2) to 3.057(2) Å. C···O distances between T-shape arranged CO 2 are in the range of 2.478(1) to 3.132(1) Å and that between π – π interacted CO 2 is 2.741(2) Å (carbon, black; hydrogen, light grey; oxygen, red; vanadium, light blue; interactions between CO 2 and frameworks are shown in green dashed line; interactions between adsorbed CO 2 molecules are shown in pink dashed line). ( e ) Binding sites for adsorbed CO 2 within MFM-300(V III ). ( f ) Binding sites for CO 2 within MFM-300(V IV ) (red and dark yellow balls indicate the centre of the corresponding binding site). Full size image The site occupancy of adsorbed CO 2 molecules was obtained by free refinement against the NPD data ( Table 2 ). At a CO 2 loading of 1.4 CO 2 /V, the occupancies of CO 2 I and CO 2 II are found to be 0.82 and 0.29, respectively. As the CO 2 loading was increased to 2.0 CO 2 per V, the occupancy of CO 2 I increased slightly to 0.99, suggesting saturation of site I, while the occupancy of CO 2 II almost doubled from 0.29 to 0.52. This result indicates that site I which contacts with the hydroxyl group directly is the preferred location for adsorbed CO 2 molecules at low surface coverage. The CO 2 molecules occupying site I have a sequential effect on the population of site II, modulated by the intermolecular dipole interaction. Table 2 Occupancy of adsorbed CO 2 molecules at different loading from the refinement against NPD data * . Full size table In contrast, the NPD pattern of CO 2 -loaded MFM-300(V IV ) shows a change in the space group from I 4 1 22 to P 4 1 22 as indicated by the appearance of Bragg peaks ( hkl , h + k + l =2 n +1), which are systematically absent in I 4 1 22 ( Supplementary Fig. 19 ). Nevertheless, the framework skeleton remains the same as that of MFM-300(V III ) and of the single crystal structure of bare MFM-300(V IV ) with four independent binding sites (I′, II′, III′ and IV′) for adsorbed CO 2 molecules being determined for CO 2 -loaded MFM-300(V IV ). Most notably, the CO 2 molecule at site I′ within MFM-300(V IV ) is rotated by 90° (compared with that in MFM-300(V III )) with respect to the bridging O 2- group and is thus side-on to the O 2- centre. It is thus sandwiched within a cleft between two phenyl rings of adjacent ligands, resulting in a highly translationally hindered site owing to the geometrical confinement ( Fig. 5b ). The linear CO 2 points to the plane of two phenyl rings with an distance of 3.069(2) and 3.146(3) Å. To our best knowledge, CO 2 binding between two phenyl rings in a ‘sandwich’ mode has not previously been experimentally observed. The CO 2 molecule at site II′ is disordered over two orientations, forming contacts to the aromatic hydrogen atoms ( =2.666(2) Å). CO 2 molecules at sites III′ and IV′ are close to the carboxylate group of the ligand with the distance ranging from 2.843(2) to 3.057(2) Å ( Fig. 5d ). In the absence of strong interactions to the MOF host, adsorbed CO 2 molecules in MFM-300(V IV ) interact between each other with short C···O distances in the range of 2.478(1) to 3.132(1) Å, and the overall packing of CO 2 in MFM-300(V IV ) is more close to the dry ice structure compared with that in MFM-300(V III ), suggesting the presence of stronger intermolecular dipole interactions in MFM-300(V IV ) ( Supplementary Fig. 20 ). Refinement of the site occupancies suggests that 20 and 10% of adsorbed CO 2 resides at site I′ and II′, respectively, at a loading of 1.4 CO 2 per V, much lower than that (60%) for the corresponding position (site I) within MFM-300(V III ) at the same CO 2 loading. This leads to 70% of adsorbed CO 2 molecules residing on sites III′ and IV′, showing a dipole interaction with the carboxylate oxygen centres, clearly suggesting that these sites (III′ and IV′) now become the primary binding sites in MFM-300(V IV ) in the absence of the hydroxyl proton. The location of adsorbed CO 2 molecules have been determined in a number of MOF systems that primarily contain open metal sites (e.g., HKUST-1 (ref. 33 ) and MOF-74 (ref. 23 )) or pendent functional groups (e.g., amine group [24] and hydroxyl group [26] ). These studies suggest that the open metal sites or functional groups in the pore have a specific role in CO 2 binding to the localized environment; their effects upon CO 2 binding on a macroscopic level are however generally overlooked. The present study of MFM-300(V III/IV ) offers a comprehensive understanding of the effect of functional groups in CO 2 binding. It is found that the hydroxyl proton plays a significant role in CO 2 binding, not only to its localized environment but also to those CO 2 molecules residing in the centre of the pore. Thus, the overall arrangement and packing of CO 2 molecules in the extended channel of these two materials are distinct with different site populations [60/40 for Site I/II in MFM-300(V III ) vs 30/70 for Sites I′+II′/III′+IV′ in MFM-300(V IV )]. Structural analysis by DFT calculation The structures for CO 2 -loaded MFM-300(V III ) and MFM-300(V IV ) have also been optimized by DFT calculation at the loading of 2CO 2 per V. The optimized structural model of MFM-300(V III )·4CO 2 shows excellent agreement with that obtained from NPD experiment, confirming the end-on model of adsorbed CO 2 molecules interacting to the hydroxyl groups ( =2.076 Å, Fig. 5e and Supplementary Fig. 21a ). In contrast, for MFM-300(V IV ), the calculated structure model does not show the ‘sandwich’ mode of adsorbed CO 2 between two phenyl rings as seen in the NPD model. This is probably because that the CO 2 -loaded MFM-300(V IV ) system has a less distinct energy minimum than the V III material, that is, the rotation/translation of adsorbed CO 2 molecules can occur more readily in MFM-300(V IV ), leading to a series of similar structural models with close energy minimum in the calculation. That said, the change of the overall arrangement and packing of CO 2 molecules in the pore has been successfully predicted by DFT calculations on going from MFM-300(V III ) to MFM-300(V IV ), consistent with the presence of weaker CO 2 –host and stronger CO 2 –CO 2 binding interaction in MFM-300(V IV ) ( Fig. 5f and Supplementary Fig. 21b ). Analysis of CO 2 binding via inelastic neutron scattering Understanding the change in dynamics upon adsorption of CO 2 within these porous hosts can provide fundamental insight into the formation of multiple supramolecular contacts (e.g., hydrogen bond and intermolecular dipole interactions) with the adsorbed gas molecules. INS is a powerful neutron spectroscopic technique that is particularly sensitive to the dynamics of hydrogen atoms owing to the exceptionally large cross-section for that isotope and is therefore used here to investigate the vibrational states of hydrogen bonded systems. Comparison of the INS spectra of the bare MFM-300(V III ) and MFM-300(V IV ) samples shows a number of differences ( Fig. 6 and Supplementary Fig. 22 ). The most significant change is the absence of the –OH out-of-plane bending mode at 47 meV and disappearance of a series of hydroxyl deformation modes between 40 and 70 meV in MFM-300(V IV ), confirming the deprotonation of the bridging hydroxyl group upon oxidation. The peaks corresponding to the C–H wagging/bending modes (80–167 meV) remain the same between these two samples. Calculated INS spectra for these two MOFs by DFT were found to be in good agreement with the experimental INS data ( Supplementary Figs 23 and 24 ). On addition of CO 2 in MFM-300(V III ), all peaks shift slightly to higher energy, indicating a stiffening effect of the host–guest lattice. Importantly, increases in intensity were observed for the peaks at 48 and 118 meV, indicating the change of the vibrational motion of both –OH and –CH groups upon CO 2 binding, consistent with the formation of hydrogen bonds and supramolecular interactions as observed in the NPD and DFT models ( Fig. 6c ). This is further confirmed by the difference spectrum, and significantly these changes are in excellent agreement with the calculated difference INS spectrum ( Fig. 6d ). In contrast, addition of CO 2 in MFM-300(V IV ) is accompanied by changes of the peak intensity at 32, 85, 117 and 158 meV, corresponding to the distortion of the MOF lattice, distortion of the phenyl rings, deformation of the phenyl ring and in-plane C–H bending modes, respectively. This result confirms unambiguously that the phenyl ring and –CH group now become the primary binding site for adsorbed CO 2 in MFM-300(V IV ), in excellent agreement with the NPD results. These changes of the INS peaks are successfully predicted from the DFT calculations with an exceptionally high degree of consistency ( Fig. 6f ). Thus, the INS results have confirmed (i) the deprotonation of the bridging hydroxyl group occurs on going from MFM-300(V III ) to MFM-300(V IV ); (ii) in MFM-300(V III ), both –OH and –CH are active binding sites for adsorbed CO 2 via formation of hydrogen bonds; (iii) in MFM-300(V IV ), the –CH and phenyl groups are the active binding sites for adsorbed CO 2 via formation of supramolecular contacts. These observations are consistent with the NPD/DFT studies and confirm the significant effects of bridging hydroxyl groups on guest binding in MFM-300(V III ). It is widely accepted that introduction of pendent functional groups into the pores of MOFs offers accessible binding sites for guest molecules by attracting them via specific interactions. These sites often lose activity after reaching a 1:1 host–guest complex and are thus believed to have a limited role in the entire gas uptake process. Many functional groups contain hydrogen donors (e.g., –OH, –NH 2 , –OCNH–, COOH, –CH 3 ), and the direct visualization of the molecular details for host–guest binding involving potential formation of hydrogen bonds is of fundamental importance to understand the function of host–guest systems. We have reported here the synthesis and characterization of a porous material, MFM-300(V III ), and its single-crystal to single-crystal transformation via post-oxidation to give its counterpart MFM-300(V IV ). The oxidation of V centres from +3 to +4 promotes deprotonation of the bridging hydroxyl group, achieving fine tuning of the pore environment. It has been confirmed that these protons play a key role in the CO 2 adsorption (both uptakes and heats of adsorption) in adsorption experiments. A study combining NPD, INS and modelling has unambiguously determined the binding sites and structural dynamics for these CO 2 –host systems. We have confirmed that the proton on the hydroxyl group can not only attract and localize adsorbed CO 2 molecules via direct formation of hydrogen bonds but also affects the macroscopic packing and arrangement of CO 2 molecules in the extended channel. Interestingly, a form of CO 2 binding to the phenyl rings has been observed in MFM-300(V IV ) by the NPD study. Thus, this report has provided direct evidence of the role of protons for guest binding in porous MOFs and, more importantly, it suggests that the effect of the functional group (i.e., protons) goes beyond specific binding to the local site and extends to the entire pore structure. Synthesis of single crystals of MFM-300(V III )-solv A mixture of VCl 3 (0.076 g, 0.48 mmol), deionized water (5.0 ml) (degassed previously under Ar for 0.5 h), biphenyl-3,3′,5,5′-tetracarboxylic acid (0.010 g, 0.03 mmol) and hydrochloric acid (1.6 M, 1.0 ml) was transferred into a 23 ml Teflon lined autoclave, which was then charged with argon and sealed. Reaction took place at 210 °C for 3 days and afforded dark green prism-shaped crystals accompanied with colourless block-shaped crystals (which are MFM-300(V III )-solv and the re-crystallized ligand, respectively). The product was soaked in fresh N,N′ -dimethylformamide (DMF) overnight to remove re-crystallized ligand, pure MFM-300(V III )-solv single crystals (ca. 5% yield) were collected by filtration and preserved in acetone. Synthesis of bulk MFM-300(V III )-solv A mixture of VCl 3 (0.40 g, 2.55 mmol) in deionized water (10.0 ml) (degassed previously under Ar for 0.5 h), biphenyl-3,3′,5,5′-tetracarboxylic acid (0.14 g, 0.42 mmol) and hydrochloric acid (0.3 M. 2.0 ml) was transferred into a 45-ml Teflon lined autoclave, which was then charged with Ar and sealed. The reaction was heated at 210 °C for 3 days to produce MFM-300(V III )-solv as a green microcrystalline powder (90% yield). This was soaked in fresh DMF overnight, and collected by filtration and stored under acetone. Preparation of desolvated MFM-300(V III ) MFM-300(V III )-solv was placed in a Schlenk flask, which was evacuated to <1 × 10 -3 mbar at ambient temperature for 1 h, and then heated at 150 °C for overnight under vacuum. Activated MFM-300(V III ) was obtained as green powder and stored in a glovebox. An important issue in desolvating MFM-300(V III ) is to avoid oxidation. Elemental analysis for MFM-300(V III ), C 16 H 8 O 10 V 2 (found (calculated%)): C 41.4(41.6), H 1.9(1.7), N 0.0(0.0). Post-synthetic oxidation of MFM-300(V III ) to prepare MFM-300(V IV ) Single crystals or powder MFM-300(V III ) was heated under pure O 2 flow at 150 °C overnight using a tube furnace. The temperature ramping speed was set to 1.0 °C min −1 . MFM-300(V IV ) was obtained as dark purple solid that was stored under N 2 in a glovebox. Elemental analysis for MFM-300(V IV ), C 16 H 6 O 10 V 2 (found (calculated)%): C 41.5(41.8), H 1.5(1.3), N 0.0(0.0). In situ single-crystal diffraction and structure determination A single crystal of MFM-300(V III ) was selected and glued onto a MiTeGen loop with Loctite Double Bubble epoxy. This was inserted into the holder of the Advanced Light Source gas environmental cell at Beamline 11.3.1, comprising a 50 μm quartz glass tube coupled to gas handling and vacuum equipment. The cell was attached to a Bruker D8 diffractometer with a PHOTON100 CMOS detector on Beamline 11.3.1 at the Advanced Light Source equipped with an Oxford Cryosystems Cryostream 800 plus. Spheres of data were collected with λ =0.7749 Å radiation, from a channel cut Silicon [111] monochromator, at various sample temperatures and pressures. The in situ oxidation was carried out in a flow-type gas cell via flowing air through the cell that was heated at 150 °C for 2 h (see Supplementary Method for more details of structure determination). EPR measurements X-band (9.86 GHz) EPR spectra were recorded on powder samples of MFM-300(V III ) and MFM-300(V IV ) at room temperature, using a BrukerEMX Micro EPR spectrometer equipped with an X-band microwave bridge, a high-Q resonator and a 1.0 T electromagnet. The microwave frequency was measured with a built-in digital counter and the magnetic field was calibrated using a Bruker strong pitch reference sample ( g =2.0028). Modulation amplitude and microwave power used were 3 G and 2 mW, respectively. Data were analysed with the Bruker Win EPR Simfonia package. Neutron powder diffraction NPD experiments were undertaken at the WISH diffractometer at the ISIS Facility. MFM-300(V) was loaded into a 6 mm diameter vanadium sample can and outgassed at 1 × 10 −7 mbar and 100 °C for 1 day. The sample was then loaded into a liquid helium cryostat and cooled to 7 K for data collection. CO 2 gas was introduced by warming the samples to 290 K, and the gas was dosed volumetrically from a calibrated volume. The gas-loaded sample was then cooled to 7 K over a period of 2 h to ensure good mobility of adsorbed CO 2 within the crystalline structure of MFM-300(V). The sample was kept at 7 K for an additional half an hour before data collection to ensure the thermal equilibrium (see Supplementary Method for more details). Inelastic neutron scattering INS experiments were undertaken using the TOSCA spectrometer at the ISIS Facility. MFM-300(V) was loaded into an 11 mm diameter vanadium sample can and outgassed at 1 × 10 −7 mbar and 100 °C for 1 day. The sample was loaded into a helium closed cycle refrigerator cryostat and cooled to 11 K for data collection. CO 2 gas was introduced by warming the samples to 290 K, and the gas was dosed volumetrically from a calibrated volume. The gas-loaded sample was then cooled to 11 K over a period of 2 h to ensure good mobility of adsorbed CO 2 within the crystalline structure of MFM-300(V). The sample was kept at 11 K for an additional half an hour before data collection to ensure the thermal equilibrium (see Supplementary Method for more details of DFT Calculation for INS spectra). Infrared measurements of gas-loaded MFM-300(V) Infrared spectroscopic measurements of crystals of MFM-300(V III ) and MFM-300(V IV ) were carried out using a Bruker Hyperion 3000 microscope equipped with an LN 2 cooled MCT detector, coupled to a Bruker Vertex spectrometer supplied with broad band radiation from beamline B22 of the Diamond Light Source. Experiments were carried out using a Linkam FTIR600 environmental gas stage under a constant (100 cm 3 min −1 ) flow of dry He. The desolvated sample was generated in situ by heating the sample to 393 K for 2 h, and 256 scan spectra were collected at 298 K. Data availability Single crystal data of MFM-300(V III ) and MFM-300(V IV ) are deposited at Cambridge Crystallographic Data Centre (CCDC) with numbers of 1479680–1479681, and numbers of 1481144–1481147 are for CO 2 -loaded MFM-300(V) samples obtained from NPD. The data that support the findings of this study are available from the corresponding author on request. How to cite this article: Lu, Z. et al . Modulating supramolecular binding of carbon dioxide in a redox-active porous metal-organic framework. Nat. 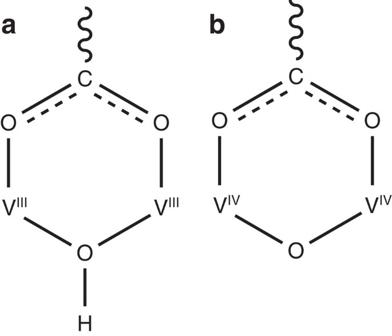Commun. 8, 14212 doi: 10.1038/ncomms14212 (2017). Publisher’s note: Springer Nature remains neutral with regard to jurisdictional claims in published maps and institutional affiliations. Figure 3: Coordination in MFM-300(VIII) and MFM-300(VIV). View of the bonding at the V centre in (a) MFM-300(VIII) (b) and MFM-300(VIV). Figure 3: Coordination in MFM-300(V III ) and MFM-300(V IV ). View of the bonding at the V centre in ( a ) MFM-300(V III ) ( b ) and MFM-300(V IV ). Full size image